Ostwald’s rule of stages governs structural transitions and morphology of dipeptide supramolecular polymers The self-assembly of molecular building blocks into nano- and micro-scale supramolecular architectures has opened up new frontiers in polymer science. Such supramolecular species not only possess a rich set of dynamic features as a consequence of the non-covalent nature of their core interactions, but also afford unique structural characteristics. Although much is now known about the manner in which such structures adopt their morphologies and size distributions in response to external stimuli, the kinetic and thermodynamic driving forces that lead to their transformation from soluble monomeric species into ordered supramolecular entities have remained elusive. Here we focus on Boc-diphenylalanine, an archetypical example of a peptide with a high propensity towards supramolecular self-organization, and describe the pathway through which it forms a range of nano-assemblies with different structural characteristics. Our results reveal that the nucleation process is multi-step in nature and proceeds by Ostwald’s step rule through which coalescence of soluble monomers leads to the formation of nanospheres, which then undergo ripening and structural conversions to form the final supramolecular assemblies. We characterize the structures and thermodynamics of the different phases involved in this process and reveal the intricate nature of the transitions that can occur between discrete structural states of this class of supramolecular polymers. The combination of supramolecular chemistry and polymer science has given rise to a diverse class of new materials [1] , [2] which bridge the gap between covalent polymers and species formed by bottom up self-assembly processes. A rich diversity of supramolecular polymer nano- and micro-structures has been described in the last two decades, including tubes, fibres, films, plates and vesicles [3] , [4] , [5] , [6] . These supramolecular materials emerge through the self-assembly of monomeric building blocks, bound together in organized structures by non-covalent interactions. The dynamic nature of such interactions within these materials can lead to molecular architectures with unique characteristics and properties, such as the ability to assemble reversibly, to undergo self-healing and to respond to external stimuli [2] , [7] , [8] . Extrinsic parameters such as pH, temperature, solvent composition and concentration have been shown to influence the molecular organization and alter the properties of these non-covalent polymers [9] , [10] , [11] . Several polymorphic self-assembly processes that lead to the formation of functional structures in biology and supramolecular chemistry have been reported [12] , [13] , [14] , [15] , [16] . The diphenylalanine (FF) structural motif and its derivatives are among the most widely studied minimal building blocks that allow the formation of ordered polymer-like assemblies at the nano-scale [17] , [18] , [19] , [20] . This class of molecular species exhibits effective self-assembly properties, and has been shown to generate a rich variety of ultrastructures, with functional physical and chemical properties, including piezoelectricity [21] , [22] , luminescence [23] and robust mechanical characteristics [24] , [25] , [26] , [27] , [28] , [29] . Moreover, it is becoming increasingly clear that the ability to control the structures of self-assembled peptides at interfaces has great potential for a multitude of future applications [30] . Polymorphism in such polymers can be influenced by the careful choice of solution conditions [11] , [31] , [32] , [33] . For instance, it has been shown that N-(t-butoxycarbonyl) -L-Phe-L-Phe-COOH (Boc-FF) can undergo self-assembly into structurally distinct states on the nanometer length scale as a result of variations in the solvent composition in which the process occurs. When assembled in aqueous solution, for example, Boc-FF forms tube-like structures that display axial hollow cores, while spherical structures are formed in a 50:50 (v/v) water–ethanol solution [33] , [34] . Whereas the crystalline tubular structures formed by Boc-FF in water reveal structural similarities to the highly ordered species formed by FF under similar conditions, the spherical assemblies, formed under certain preparation conditions, display only a partial degree of crystalline order [35] . Studies of the mechanical properties of these spheres have revealed a remarkable metallic-like point stiffness of up to 885 Nm −1 and a Young’s modulus of up to 275 GPa (ref. 35 ), reflecting the very high degree of rigidity that can be achieved by supramolecular assemblies. In the present study, we provide a description of the assembly pathways of Boc-FF supramolecular polymers and show that their formation proceeds through metastable phases displaying spherical and fibrillar morphologies, into the final stable state of crystalline tubes [34] . Furthermore, we characterize the free energies of the intermediate phases and show that these metastable phases form in order of increasing stability, and are therefore governed by Ostwald's rule of stages [36] . Such spherical, filamentous and fibrillar morphologies are commonly observed for supramolecular structures from peptides [37] , [38] , [39] , although the characterization of structural transitions linking such phases has heretofore remained elusive. These results open up the possibility of controlling the morphology of supramolecular polymers through kinetic as well as thermodynamic means. Phase behaviour We initiate the self-assembly of Boc-FF into nanostructures by generating supersaturated solutions of the precursor monomer in an ethanol and water mixture. The lower solubility of Boc-FF in water relative to ethanol enables supersaturation to be achieved by diluting a concentrated solution of the dipeptide in ethanol through the addition of water. We probe the phase behaviour of the dipeptide system, as shown in Fig. 1a , by varying systematically the ratio of water to ethanol, from pure ethanol to 10% ethanol in water, and also by varying the concentration of the dipeptide from 0.2–10 g l −1 , using 96-well plates, sealed to avoid evaporation and allowed to equilibrate for 1 h prior to measurement. Our results show a clear change in the relative stabilities of the self-assembled phases of this supramolecular polymer system as a function of the different variables. At the lowest concentration of Boc-FF (0.2 g l −1 ) and the highest ratios of water to ethanol, we detect self-assembled tubular structures by light microscopy; as the concentration of Boc-FF is increased, however, two distinct populations of structures are identified, spheres and tubes, in varying ratios. 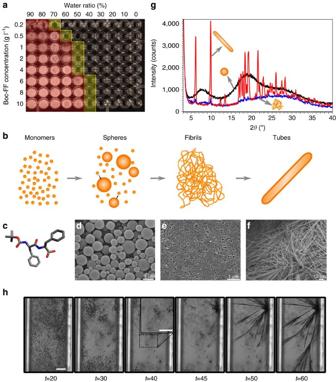Figure 1: Morphological characterization of Boc-FF self-assembly. (a) Phase diagram based on experiments using 96-well plates in which an isotropic solution forms first spheres (yellow) and then tubes (red) as water of ethanol ratios (horizontaly) and the Boc-FF concentration (vertically) are varied. (b) Schematic depiction of the phase transition observed in the Boc-FF system over time. (c) Schematic molecular structure of Boc-FF. (d–f) Aliquots of Boc-FF with a final concentration of Boc-FF in 10% ethanol and water solution were collected at 2, 40 and 60 min and left to dry on glass slides. (d) Boc-FF spheres seen after 2 min of the initiation of the assembly reaction (scale bar, 1 μm). (e) Boc-FF filaments forming gel-like matrices seen after 40 min (scale bar, 1 μm). (f) Boc-FF tube formation seen after 60 min (scale bar, 10 μm). (g) Powder X-ray spectra from each isolated structural type, 2θ3–40°. (h) Bright field images of Boc-FF spheres at 1:10 ethanol–water solution, which were transferred into a glass capillary and then sealed, were taken at 20, 30, 40, 45, 50 and 60 min. The spheres that are visible over 20 min, are seen to disassemble slowly, giving rise to fibrillar assemblies at 30 and 40 min time points. This filamentous assembly (insert, scale bar 40 μm) is shown at a magnified scale to allow visualization of the assembled fibrils. The filaments then disassemble, and tubes are shown to grow from centres found in the vicinity of the fibrillar assemblies at 45, 50 and 60 min. Scale bars, 50 μm. Figure 1: Morphological characterization of Boc-FF self-assembly. ( a ) Phase diagram based on experiments using 96-well plates in which an isotropic solution forms first spheres (yellow) and then tubes (red) as water of ethanol ratios (horizontaly) and the Boc-FF concentration (vertically) are varied. ( b ) Schematic depiction of the phase transition observed in the Boc-FF system over time. ( c ) Schematic molecular structure of Boc-FF. ( d – f ) Aliquots of Boc-FF with a final concentration of Boc-FF in 10% ethanol and water solution were collected at 2, 40 and 60 min and left to dry on glass slides. ( d ) Boc-FF spheres seen after 2 min of the initiation of the assembly reaction (scale bar, 1 μm). ( e ) Boc-FF filaments forming gel-like matrices seen after 40 min (scale bar, 1 μm). ( f ) Boc-FF tube formation seen after 60 min (scale bar, 10 μm). ( g ) Powder X-ray spectra from each isolated structural type, 2 θ 3–40°. ( h ) Bright field images of Boc-FF spheres at 1:10 ethanol–water solution, which were transferred into a glass capillary and then sealed, were taken at 20, 30, 40, 45, 50 and 60 min. The spheres that are visible over 20 min, are seen to disassemble slowly, giving rise to fibrillar assemblies at 30 and 40 min time points. This filamentous assembly (insert, scale bar 40 μm) is shown at a magnified scale to allow visualization of the assembled fibrils. The filaments then disassemble, and tubes are shown to grow from centres found in the vicinity of the fibrillar assemblies at 45, 50 and 60 min. Scale bars, 50 μm. Full size image Monomer to sphere transition To obtain insights into the assembly pathways of these different phases, we monitor the time evolution of the system at different water to ethanol ratios, starting from a solution containing a fixed value of 10% (v/v) ethanol in water. Initially, dilution into water of a stock solution of Boc-FF in ethanol results in opaque, milky solutions. After further incubation for ca . 30 min, however, the solutions become clearer and filamentous aggregates are observed, while at the endpoint of the experiment, achieved after ca . 60 min, the tubes can be detected by light microscopy, as displayed by the scheme in Fig. 1b . Figure 1c–f shows the structure of the Boc-FF monomer and high-resolution scanning electron microscope (HR-SEM) images of the three distinct types of structures identified in the course of this reaction. The progressive formation of these different types of structures coincides with changes in the optical appearance of the solutions over time. Thus, while the measured turbidity of the solutions increases by a substantial degree due to light scattering from the spheres present, the level of turbidity subsequently decreases as more compact nano-fibrillar or filamentous structures forming gel-like assemblies emerge; these species are ultimately observed to convert to tubes ( Fig. 1d–f ). We then isolate samples of the three different phases, and record powder X-ray diffraction patterns for each of them; the results are presented in Fig. 1g . The spherical species, after removal of solvent, show a diffraction pattern typical of amorphous materials, with two broad halos. The diffraction pattern of samples of the gel phase, however, differs considerably from that of the spherical species, with flattening and partial resolution of the broad peaks centred at 2 θ =8° and 19°. While the gel itself can be seen to be devoid of ordered crystallinity, the further peaks of a low amplitude in the fibrillar phase are likely to be due to the presence of small quantities of tubular crystals, see below. The diffraction patterns demonstrate that the spherical and filamentous structures are both largely amorphous in nature, but that the short-range order present in each type of structure is different. The tubular structures are, however, highly crystalline as shown by their diffraction pattern which exhibits distinct sharp peaks with high intensity. We next seek to follow the spatial and temporal appearance and conversion of the structural phases. To this effect, time-lapse optical microscopy measurements are conducted on supercritical solutions of Boc-FF, sealed in glass capillaries to prevent evaporation. The data in Fig. 1h show that the spheres initially present in such systems are progressively replaced by fibrillar species after incubation in a glass capillary for ca . 30 min. The fibrillar phase is found to be localized initially at a single point, seen as filamentous aggregates by light microscopy, but is observed to spread progressively in space. Dissolution of the spheres is observed to occur in the vicinity of this growing network of fibrils, resulting in the quantitative conversion over time of Boc-FF from the spheres to the filamentous form of self-assembled structures. Shortly after the emergence of the filamentous phase, thicker tubular structures are observed to form rapidly (see Supplementary Movie 1 ). Tube nucleation is seen to be spatially correlated with the presence of filamentous aggregates of the fibrillar phase, which are visible in the Supplementary Movie 1 and in Fig. 1h . Moreover, as can be observed in Fig. 1g , the X-ray diffraction baseline pattern of both fibrils and tubes is similar, indicating a structural relationship between the fibrillar and tubular species. These observations suggest, therefore that the tubular phase initially forms from the fibrillar phase. Moreover, while fibrillar aggregates can be detected in the vicinity of the locations where tube growth initiates ( Fig. 1h ), the average diameter of individual fibrils is about 30 nm ( Fig. 1e ), and is not readily observed by light microscopy. We note that the changes are consistent with a mechanism whereby monomers detach from structures of one type, diffuse in solution and are incorporated in another type of supramolecular assembly. In particular, the sphere phase is observed to be depleted as the fibrillar and tubular phases grow in space. The sequential formation of multi- branched tubular structures, shown in Fig. 1h suggests that the proliferation of the tubes is driven by secondary nucleation [40] , [41] , [42] , [43] and subsequent growth of new tubular structures occurs from the surfaces of existing tubes. Nucleation is a rare event and, as such, is expected to be statistically suppressed in small volumes [44] , [45] , [46] . To test whether or not the emergence of the tubular phase of the self-assembly of Boc-FF scales with system volume, we compare results from bulk experiments with those obtained in microdroplets, where the aqueous solutions are encapsulated as emulsions in an immiscible oil phase (see methods). The phase transition from spheres to tubes occurs reproducibly within 30–45 min in droplet volumes approaching those of the bulk solution (average droplet volume=7 nl), yet when encapsulated in picolitre droplets (average droplet volume=300 pl), the spheres are stable for significantly longer periods of time without undergoing a phase transition ( Fig. 2a ). Indeed, in the droplets with the largest volumes the phase transition from spheres to tubes is detectable after 30–45 min, in the low volume microdroplets the spheres remain present at all times monitored in our experiments ( Fig. 2b ). These observations show that the formation of tubes is significantly suppressed in small volumes and therefore has the characteristics of a nucleated process [45] . 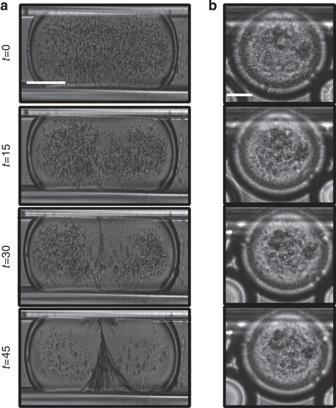Figure 2: Phase transition of Boc-FF spheres after spatial confinement over time. (a) Bright field images of phase transition from spheres to tubes occurring in a droplet with volume of 7 nl over the course of 45 min. Scale bar, 100 μm. (b) Bright field images show the stability of the spherical phase over the same time period under volume confinement (droplet volume 300 pl). Scale bar, 25 μm. Figure 2: Phase transition of Boc-FF spheres after spatial confinement over time. ( a ) Bright field images of phase transition from spheres to tubes occurring in a droplet with volume of 7 nl over the course of 45 min. Scale bar, 100 μm. ( b ) Bright field images show the stability of the spherical phase over the same time period under volume confinement (droplet volume 300 pl). Scale bar, 25 μm. Full size image To probe the transition of the isotropic monomer solution into the spherical structures, we monitor the assembly of polymeric structures by measuring the concentration of free Boc-FF in solution by ultraviolet–visible spectroscopy ( Fig. 3a ). Despite varying the initial concentration of initial Boc-FF monomers by a factor of 5, the concentrations of the soluble form of the dipeptide measured after incubation for 12 min are identical to within 3%. These results indicate rapid primary nucleation of free monomers into spheres, which serve as the main monomer sink after the solution has achieved supersaturation. 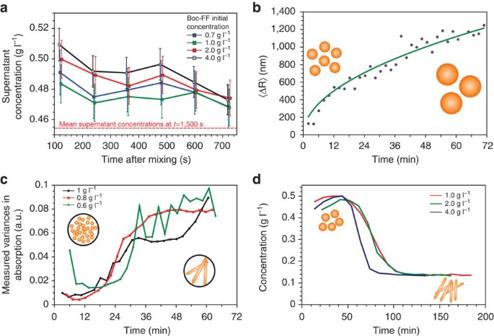Figure 3: Quantitative analysis of Boc-FF sphere maturation and tubular phase formation. (a) Decrease in supernatant concentration over time, measured spectroscopically from the filtrate at 257.6 nm. Error bars are calculated from the polydispersity index (n=5). (b) Changes in sphere radius by DLS measurements over 60 to 780 s post mixing. The linearity suggests an Ostwald ripening process taking place over time. (c) Change in anisotropy with time. The results show that all samples nucleate in a short time window of ~10 min after initiation of the reaction, the relative rapidity of this onset being due to agitation of the samples through repeated rapid motions during the well scanning operation. (d) NMR analysis of changes in the free Boc-FF monomer concentration as the phase transition proceeds over time. Figure 3: Quantitative analysis of Boc-FF sphere maturation and tubular phase formation. ( a ) Decrease in supernatant concentration over time, measured spectroscopically from the filtrate at 257.6 nm. Error bars are calculated from the polydispersity index ( n =5). ( b ) Changes in sphere radius by DLS measurements over 60 to 780 s post mixing. The linearity suggests an Ostwald ripening process taking place over time. ( c ) Change in anisotropy with time. The results show that all samples nucleate in a short time window of ~10 min after initiation of the reaction, the relative rapidity of this onset being due to agitation of the samples through repeated rapid motions during the well scanning operation. ( d ) NMR analysis of changes in the free Boc-FF monomer concentration as the phase transition proceeds over time. Full size image Ostwald ripening Following the rapid initial formation of spheres, these structures are observed to change size progressively over a timescale of minutes ( Fig. 3b ). This behaviour can be attributed to Ostwald ripening [47] , [48] , a process in which monomers preferentially re-solvate from smaller species, where the fraction of solvent-exposed sites is larger, and are re-incorporated in larger aggregates. For processes where monomer addition to the growing aggregates is limited by surface processes rather than diffusion in the solution, the average particle size changes according to the relationship [49] , [50] ‹ R ( t ) 2 ›−‹ R (0) 2 › ∝ t , where t is the time and R ( t ) is the radius of the particle at time t . The average particle size is therefore expected to change with the root of incubation time, and the results, closely agreeing with this prediction (green line), are shown in Fig. 3b . Moreover, dynamic light scattering (DLS) measurements indicate that the average sizes of the spheres increase without being accompanied by a corresponding decrease in the concentration of the monomeric dipeptide ( Fig. 3a ). Thus, the change in the average particle size cannot be accounted for by depletion of monomer from solution but rather emerges as a result of a redistribution of mass between the particles through Ostwald ripening [51] , [52] . To characterize the possibility of tube formation from coalescence between spheres, we evaluate the strength of the electrostatic repulsions between individual particles by measuring their ζ -potential (see Methods). We found that over the first 5 min after formation, the average zeta-potential of the system was observed to remain constant within experimental error at −73±2 mV, a value which represents a repulsive electrostatic barrier larger than k B T (25 mV) for an elementary charge and is thus indicative of electrostatic stability with respect to coalescence [52] . This large value indicates that the spheres form a highly stable colloidal suspension and that coalescence of the particles is strongly suppressed. Sphere-to-tube transition Ostwald ripening processes can result in the internal rearrangement and recrystallization of structures formed in kinetically driven self-assembly processes [54] . To probe for the possibility of such a process, kinetic assays for evaluating the rate of sphere-to-tube rearrangement are performed through spatially resolved optical density measurements monitoring the variance as a function of time between the absorbance at nine points separated by a distance of 1.2 mm on a square grid. The optical density of a suspension of spheres is found initially to be, on average, uniform throughout the sample; however, a transition from this uniform density of a suspension of micron sized spheres to a markedly inhomogeneous suspension of the much larger tubes is observed to take place over time, Fig. 3c . To follow the kinetics of this process in more detail, we measure by means of Nuclear Magnetic Resonance (NMR) spectroscopy the time evolution of the concentration of monomeric Boc-FF in the suspension of the tubes. The data in Fig. 3d show the change in the intensity of the methyl 1 H resonance of Boc-FF when the dipeptide is solubilized in 90% H 2 O-10% EtOD as a function of time for three different initial monomer concentrations. Once spheres or tubes form, the intensity of the free Boc-FF signal is of a similar order of magnitude and is observed to be independent of the starting concentration. This observation suggests that these concentrations represent the (pseudo-)equilibrium solubilities of Boc-FF with respect to the spherical or tubular phases. In the presence of the spheres, the free monomer concentration is measured to be 0.52 g l −1 , while at the end of the reaction, when all the spheres convert into tubes, a concentration of 0.14 g l −1 is measured. Thus, the free monomer concentration in the solution is seen to be reduced as the assembly of further, more stable structures, occurs ( Fig. 3d ). This observation clearly indicates that formation of the tubular state depletes the concentration of free monomers in solution, along with the incorporation of monomers which have been incorporated in the previous, less stable structures, which are released to the solution by their disassembly. To gain additional insight into the thermodynamic characteristics of the phase transition between spheres and tubes, we monitor the phase transition at a peptide concentration of 0.75 gl −1 by differential scanning calorimetry (DSC), in constant temperature mode. Using this method, we follow the exothermic or endothermic processes leading to, and occurring at, the phase transition between spheres and tubes by comparison of the heat changes taking place in a 1:10 ethanol to water solution containing 0.75 g l −1 Boc-FF compared with a control solution devoid of the peptide. The data show a release of heat at a time corresponding to the observed timescale for the transition from spheres to tubes by microscopy analysis. This observation indicates that the transition from spheres to tubes is exothermic in the temperature range investigated (10–20 °C), with a corresponding enthalpic change Δ H s,t =−21±2.1 kJ mol −1 , and that the apparent heat capacity of the reaction is small ( Fig. 4a ). 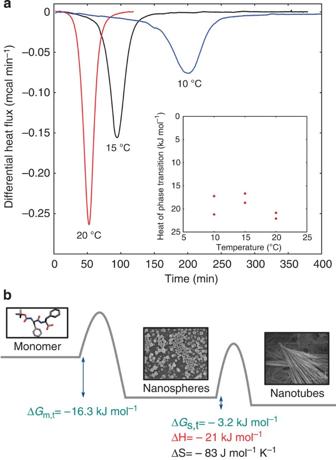Figure 4: Kinetic and thermodynamic changes during the phase transition. (a) Differential scanning calorimetry measurements of the transition from spherical to tubular structures. Plotted is the differential heat flux to maintain the sample cell and the reference cell at the same temperature. Inset: the integrals of the data in the main figure represent the total amount of heat that is released during the phase transition. It can be seen that ΔHs,tdoes not depend strongly on temperature in the investigated interval. (b) Schematic free energy diagram for the Boc-FF transition from the metastable state of the spheres to that of the stable state of the tubes. Figure 4: Kinetic and thermodynamic changes during the phase transition. ( a ) Differential scanning calorimetry measurements of the transition from spherical to tubular structures. Plotted is the differential heat flux to maintain the sample cell and the reference cell at the same temperature. Inset: the integrals of the data in the main figure represent the total amount of heat that is released during the phase transition. It can be seen that Δ H s,t does not depend strongly on temperature in the investigated interval. ( b ) Schematic free energy diagram for the Boc-FF transition from the metastable state of the spheres to that of the stable state of the tubes. Full size image Of further significance is that our results show that the concentration of monomer in equilibrium with the tubular phase is lower than that found in equilibrium with the spheres ( Fig. 3d ), indicating that the thermodynamic stability of the tubular phase is higher than that of the spherical phase, and hence the transition is governed by Ostwald’s rule of stages. This rule predicts that a system evolves through a series of phase transitions, each successive phase is characterized by the smallest loss of free energy relative to its predecessor before finally reaching the most thermodynamically stable form. This rule has been shown to apply to a range of polymer systems in both experimental [55] , [56] and computational studies [57] , [58] , yet few examples of this phenomenon have been reported for supramolecular peptide polymers [59] . The critical concentration with respect to the results observed by the NMR experiments ( Fig. 3d ) of both the spherical and tubular phases, 0.52 and 0.14 g l −1 , respectively, can be converted to the Gibbs free energy Δ G of each of the stages, through chemical thermodynamics: where β =( k B T ) −1 , T is the absolute temperature, k B is the Boltzmann constant. The Gibbs free energy difference between the monomeric and spherical states is Δ G m,s , as calculated from the solubility equilibrium constant is found to be −16.3 kJ mol −1 , and between the monomeric and tubular states of Boc-FF, Δ G m,t , is calculated to be −19.6 kJ mol −1 , showing a progressive decrease in system free energy during the formation of the thermodynamic product, the tubes ( Fig. 4b ). From these values, the free energy difference between the spherical and tubular states can be calculated to be −3.2 kJ mol −1 . In combination with the calorimetry measurements, this free energy can further be decomposed into the entropic and enthalpic contributions ( Fig. 4b ). In this transition from amorphous spheres to crystalline tubes, ( Fig. 4a ), the entropy change is unfavourable. As can be seen from the measured values of the thermodynamic parameters, this entropy loss is compensated by a significant enthalpic contribution to yield an overall favourable Gibbs free energy. The present work, therefore, connects three structurally distinct supramolecular phases through the rule of stages, and hence by expanding our understanding of the effect of solution composition [60] and other variables, opens up the possibility of controlling the morphology of supramolecular polymers through kinetic rather than conventional thermodynamic means. In conclusion, we demonstrate that a multi-step phase transition process underlies the supramolecular assembly of Boc-FF peptides, and that this transition exhibits a rich diversity in structural phases, from spheres to tubes. The results indicate that the spheres, previously envisioned as distinct end-products of a solvent-induced self-assembly process [34] , [35] , can undergo a second self-assembly event, resulting in the formation of tubes. The time course observable for this transition reveals that, while the species with spherical and fibrillar morphologies are transient, the tubular structures emerge as the most stable thermodynamic product, undergoing no further structural transition under the conditions studied here. Variation of the conditions under which these three distinct morphologies are formed, particularly the solution composition and the monomer concentration, have enabled us to identify the exact conditions under which specific structural phase transitions take place, and to characterize the kinetic and thermodynamic determinants governing these processes. The results of these studies indicate that the spheres initially form through a rapid condensation in the solution phase, and then undergo a process of Ostwald ripening over a longer timescale, and finally convert, in an exothermic reaction, into the thermodynamically most stable form of tubes. The understanding of the steps of this coordinated process described in this study, allows the elucidation of the molecular mechanism, leading to the formation of specific species. Our data suggest that as the direct coalescence of spheres is unlikely in view of the value of their ζ -potential, other transition mechanism may occur. The suppression of this mechanism in small volumes indicates that it is likely to be a nucleated process; moreover, the spatial development of the fibrillar phase leads to the depletion of the spherical phase, suggesting that the fibrils grow through monomer addition and that thermodynamic stability of the monomers in the fibrillar phase is greater than in the sphere phase; these observations suggest a thermodynamic driving force for the formation of the intermediate fibrillar phase. Interestingly, examples of transitions from amorphous aggregates into ordered tubular structures have been reported in the field of inorganic polymers [61] , [62] . While it has not been demonstrated that such systems follow the mechanism that we elucidate here for supramolecular polymer phase transitions, there are similarities in the overall process. The condensation and reorganization process described here may be analogous to that of the molecular reorganizations observed in the self-assembly of soluble proteins into amyloid fibrils, where a variety of intermediate species, including different types of oligomeric species have been observed [57] , [63] . The results described here for this archetypical supramolecular polymer, Boc-FF, exemplify the multi-step self-assembly processes, leading to the formation of supramolecular structures. A molecular level understanding of such processes opens up the possibility of the quantitative control of the end product of self-assembly, and thus allows the utilization of self-assembling dipeptide building blocks to yield supramolecular polymers with a wide range of future applications. Phase behaviour N-(t-butoxycarbonyl) -L-Phe-L-Phe-COOH (Boc-FF, Bachem) stock solutions were prepared in absolute ethanol and then diluted in the required ratios in double distilled water, forming an array of peptide concentrations and solvent compositions. The structural morphologies of the resulting species were then determined by bright field microscopy and SEM observations. In all following experiments, Boc-FF stock solution in ethanol was diluted to form 10% (v/v) ethanol in water solution and phase behaviour was monitored by the following methods. Isolation of different phases Suspensions of Boc-FF spheres were prepared by mixing of 1 part in 10 by volume stock solution of its monomers into ddH2O followed by gentle mixing. The tubular phase was isolated by the vigorous agitation of this suspension or by allowing this solution to stand for 1 h. The fibrillar phase was isolated by centrifugation of suspensions of spheres at 4 °C and the separation of the supernatant. The supernatant was stored at 4 °C for 15–20 min and was then flash frozen with liquid nitrogen and dried under reduced pressure. ultraviolet–visible spectroscopy Ten-millilitre aliquots of a suspension of Boc-FF were prepared as described above and allowed to stand in a syringe. At 2-min intervals, the suspension was gently agitated and 1.5 ml was pushed through a 0.22 μm syringe filter (Millex Ultrapore, PVDF membrane). The concentration of Boc-FF in these aliquots was determined from the difference in specific absorbance at 257.6 nm and a baseline at 300 nm using Cary-Varian 400 spectrophotometer running WinUV software. The spectral bandwidth was 1.0 nm. Dynamic light scattering One millilitre suspensions of Boc-FF were prepared as described above, and 100 μl aliquots were introduced into a low volume DLS cell. The refractive index was estimated to be 1.450 and the absorbance to be 0.001. The dispersant viscosity was taken to be 1.538 cP, and the dispersant refractive index as 1.339. Size measurements were made at 20 °C using a Malvern Zetasizer Nano ZSP (Malvern Instruments, Malvern, UK). ζ -potential measurements were performed in a Malvern disposable folded capillary cell the same parameters as above and with the additional specification of a dispersant dielectric constant at ε r =69.4. Measurements were averaged over the first 5 min after sample preparation. Differential scanning calorimetry DSC experiments were performed with a VP-DSC instrument (GE Healthcare, Amersham, UK) in isoscan mode at a constant temperature of 10–20 °C. The reference cell was filled with 10% by volume of an ethanol solution in water, and the sample cell was filled with a sample of Boc-FF spheres, prepared immediately prior to its introduction into the instrument by adding 10% by volume of a 7.5 g l −1 Boc-FF stock solution in ethanol into water. For experiments conducted below room temperature, the water was pre-cooled and the DSC instrument was pre-set to a temperature of 4 °C below that at which the experiment was to be performed, to minimize the time between sample introduction and the beginning of each measurement. Baseline measurements were subtracted from the reaction measurement, and the area of the exothermic peak integrated to yield the enthalpy of transition. Microdroplet formation Microfluidic channels were fabricated in polydimethylsiloxane (Dow Corning, Midland, MI, USA) using SU8 on silicon masters and standard soft lithography techniques, and then plasma bonded to glass slides to create sealed devices. Boc-FF stock solutions in ethanol were mixed on chip to form a solution of 10% (v/v) ethanol in water, and microdroplets were formed in an oil phase of Fluorinert FC-40 (Sigma-Aldrich, Gillingham, UK) and 2.0% (ww) block-copolymer surfactant. Syringe pumps (Cetoni GmbH, Korbussen, Germany) were used to control the flow of fluids, and the microdroplets were immediately inserted into rectangular glass capillaries (CM Scientific, Silsden, UK) sealed and then observed under bright field microscopy as a function of time. High-resolution scanning electron microscopy Samples of Boc-FF solutions at 1:10 ethanol/water ratios at various time points after the initiation of self-assembly were placed on glass slides and were left to dry at room temperature. Samples were then coated with Cr and viewed using a JSM-6700 field-emission HR-SEM (Jeol, Tokyo, Japan), equipped with a cold field emission gun, operating at 1 kV. Nuclear magnetic resonance spectroscopy NMR data were acquired using a BRUKER Avance 700 Ultrashield spectrometer equipped with TXI Cryoprobe. Samples of the Boc-FF peptide were dissolved in 100% EtOD and then diluted to form solutions of 10% (v/v) ethanol in H 2 O. One-dimensional 1 H spectra were rapidly acquired at 25 °C using 180 water-selective pulses to suppress resonances from H 2 O. NMR data were processed and analyzed using TOPSPIN. X-ray powder diffraction Samples of the spheres, gels and tubes were prepared as above and mechanically ground into fine powders. The resulting samples were placed in a flat glass sample holder and XRPD data was collected on a laboratory Philips X’Pert Pro diffractometer using Bragg-Brentano geometry. X-rays were generated using Ni-filtered Cu Kα1 radiation ( λ =1.54056 Å) generated at 40 kV and 40 mA at 298 K and a scan range of 3–60° 2 θ and a step size of 0.033° 2 θ . Continuous scans were done using the gonio scan axis, and data were analyzed using X’Pert HighScore Plus. The nano-scale ultrastructure of the spheres, fibrils and tubes was retained in the fine powders as confirmed by electron microscopy. How to cite this article: Levin, A. et al. Ostwald’s rule of stages governs structural transitions and morphology of dipepetide supramolecular polymers. Nat. Commun. 5:5219 doi: 10.1038/ncomms6219 (2014).